Transdifferentiation of lung adenocarcinoma in mice withLkb1deficiency to squamous cell carcinoma Lineage transition in adenocarcinoma (ADC) and squamous cell carcinoma (SCC) of non-small cell lung cancer, as implicated by clinical observation of mixed ADC and SCC pathologies in adenosquamous cell carcinoma, remains a fundamental yet unsolved question. Here we provide in vivo evidence showing the transdifferentiation of lung cancer from ADC to SCC in mice: Lkb1 -deficient lung ADC progressively transdifferentiates into SCC, via a pathologically mixed mAd-SCC intermediate. We find that reduction of lysyl oxidase (Lox) in Lkb1 -deficient lung ADC decreases collagen disposition and triggers extracellular matrix remodelling and upregulates p63 expression, a SCC lineage survival oncogene. Pharmacological Lox inhibition promotes the transdifferentiation, whereas ectopic Lox expression significantly inhibits this process. Notably, ADC and SCC show differential responses to Lox inhibition. Collectively, our findings demonstrate the de novo transdifferentiation of lung ADC to SCC in mice and provide mechanistic insight that may have important implications for lung cancer treatment. Lung cancer is one of the most devastating diseases worldwide with high mortality [1] . As the major lung cancer type, non-small cell lung cancer (NSCLC) is further characterized by a high degree of histopathological heterogeneity including adenocarcinoma (ADC, ~48%), squamous cell carcinoma (SCC, ~28%) and large cell carcinoma (~24%) [2] , [3] . Based on histopathological appearance and gene expression signature, it is widely speculated that these cancer subtypes arise from distinct cells of origin, for example, ADC is considered to arise mainly from alveolar epithelial cells such as type II pneumocyte, whereas SCC is from basal cells [4] , [5] . Accordingly, ADC mainly expresses type II pneumocyte marker pro-surfactant protein C (SP-C), and SCC expresses basal cell markers Trp63 ( p63 ) and Cytokeratin 5/14 ( Krt5/14 ) [6] , [7] . However, definitive evidence is not yet available in order to identify the cells of origin for either lung ADC or SCC. The mixed ADC and SCC pathology with identical genetic mutations has been frequently observed in a single lesion of human lung tumours, so called adenosquamous cell carcinoma (Ad-SCC) [8] , [9] , [10] , [11] , suggesting a monoclonality and the potential lineage transition between these subtypes. Whether there exist lineage correlation or dynamic transition between lung ADC and SCC in Ad-SCC is a fundamental yet unsolved question, not only important for a better understanding of lung cancer biology but also potentially helpful for lung cancer therapies in clinic. However, the paucity of matched clinical specimens at different stages from same patients makes it difficult to examine the dynamic transition of lung cancer; instead, this could be benefited from studies in genetically engineered mouse models of human lung cancer [12] . The tumour suppressor LKB1 encodes an evolutionarily conserved serine/threonine kinase essential for both cellular growth and metabolic homoeostasis [13] , [14] , [15] . Loss-of-function mutations of LKB1 have been observed in human lung ADC, SCC and Ad-SCC specimens [16] , [17] . Interestingly, both lung ADC and SCC with typical pathologies were consistently observed in Kras G12D , Lkb1 L/L ( Kras/Lkb1 ) mouse model [16] . It’s worth noting that the observation of lung SCC is quite unique to Kras/Lkb1 mouse model since no squamous lesion but only ADC has been observed in other models including Kras , Egfr and Kras/p53 mouse models [3] , [12] , [16] , [18] . However, it remains unknown how SCC arises in Kras/Lkb1 mouse model. Through lineage-tracing experiments and pathological analyses in Lkb1 -deficient mouse models of human lung cancer, we here show that mouse lung ADC can transdifferentiate into SCC, progressively via pathologically mixed adenosquamous cell carcinoma as an intermediate. We find that hypoxia deregulation in Lkb1 -deficent ADC results in the decrease of Lox expression as well as collagen deposition, and initiates extracellular matrix (ECM) remodelling and turns on squamous signature gene expression, which upregulates p63 expression. Interfering collagen maturation in Kras/Lkb1 mice promotes ADC to SCC transdifferentiation, while ectopic Lox expression significantly inhibits this process. Further studies show that pharmacological inhibition of Lox effectively suppresses the progression of Lkb1 -deficient ADC and promotes ADC to transdifferentiate into SCC, but has little effects upon the growth of SCC. These findings provide mechanistic insight into lung ADC to SCC transdifferentiation in mice and may have implications for future lung cancer treatment. ADC to SCC transdifferentiation in Kras/Lkb1 mouse model We first carefully monitored the progression of different subtypes of lung tumours in a group of Kras/Lkb1 mice treated with recombinant adenovirus expressing Cre recombinase (Ad-Cre). These mice were killed for histopathological analyses at a series of time points post Ad-Cre infection. At as early as 2 weeks post Ad-Cre treatment, atypical adenomatous hyperplasia (AAH) and epithelial hyperplasia were observed as the dominant types of lesions ( Fig. 1a and Supplementary Fig. 1a ). At 6 weeks post Ad-Cre treatment, papillary adenoma and ADC were evident ( Fig. 1a,b ; Supplementary Fig. 1a ). Although caution is warranted, at this stage we didn’t detect any obvious squamous lesion by pathological inspection, immunohistochemical staining and statistical analyses of SCC marker Trp63 (p63) ( Fig. 1b ; Supplementary Fig. 1b,c ). 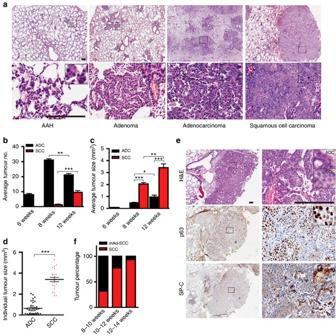Figure 1:Lkb1-deficient Lung ADC progressively transdifferentiates into SCC. (a) Representative histology for AAH, adenoma, ADC and SCC lesions inKras/Lkb1mice at a serial of time points post Ad-Cre treatment. Scale bar, 150 μm. (b,c) Quantification of average tumour number (b) and tumour size (c) per mouse for ADC and SCC inKras/Lkb1mice at 6 weeks (n=6), 8 weeks (n=12) and 12 weeks (n=8) post Ad-Cre treatment. Data are shown as mean±s.e.m.t-test, *P<0.05, **P<0.01, ***P<0.001. (d) Quantification of individual tumour size for ADC and SCC inKras/Lkb1mice at 10–12 weeks post Ad-Cre treatment.n=12, Data are shown as mean±s.e.m.t-test, *P<0.05, **P<0.01, ***P<0.001. (e) Representative mAd-SCC shown with haematoxylin and eosin staining, p63 and SP-C immunohistochemical staining on serial sections. Scale bar, 150 μm. (f) Quantification of tumour percentage for mAd-SCC and SCC inKras/Lkb1mice at indicated time points post Ad-Cre treatment.n=8 for each time point. Scale bar, 150 μm. Data are shown as mean±s.e.m.t-test, *P<0.05, **P<0.01, ***P<0.001. Only after 8 weeks of Ad-Cre treatment, we began to observe very few typical SCCs with big tumour sizes among a wide spectrum of lesions composed of AAH, epithelial hyperplasia, adenoma and ADC ( Fig 1a,b ). At an even longer time (12 weeks) post Ad-Cre treatment, the number of SCC increased concomitantly with a decrease of ADC number, while the total tumour number showed no significant change ( Fig. 1b ). Consistent with our previous study, local metastasis was detected in 3 of 19 (16%) mice at 10–12 weeks post Ad-Cre treatment and all these tumours were ADC. Figure 1: Lkb1 -deficient Lung ADC progressively transdifferentiates into SCC. ( a ) Representative histology for AAH, adenoma, ADC and SCC lesions in Kras/Lkb1 mice at a serial of time points post Ad-Cre treatment. Scale bar, 150 μm. ( b , c ) Quantification of average tumour number ( b ) and tumour size ( c ) per mouse for ADC and SCC in Kras/Lkb1 mice at 6 weeks ( n =6), 8 weeks ( n =12) and 12 weeks ( n =8) post Ad-Cre treatment. Data are shown as mean±s.e.m. t -test, * P <0.05, ** P <0.01, *** P <0.001. ( d ) Quantification of individual tumour size for ADC and SCC in Kras/Lkb1 mice at 10–12 weeks post Ad-Cre treatment. n =12, Data are shown as mean±s.e.m. t -test, * P <0.05, ** P <0.01, *** P <0.001. ( e ) Representative mAd-SCC shown with haematoxylin and eosin staining, p63 and SP-C immunohistochemical staining on serial sections. Scale bar, 150 μm. ( f ) Quantification of tumour percentage for mAd-SCC and SCC in Kras/Lkb1 mice at indicated time points post Ad-Cre treatment. n =8 for each time point. Scale bar, 150 μm. Data are shown as mean±s.e.m. t -test, * P <0.05, ** P <0.01, *** P <0.001. Full size image Although SCC appeared at a much later time point than ADC, the average tumour size of SCC was evidently bigger than that of ADC ( Fig. 1c,d ). It is more likely that these abruptly appearing SCCs are developed from those ADCs at late time point. To further confirm this, we dissected primary tumours from Kras/Lkb1 mice at 6 weeks post Ad-Cre infection, with part of them for serial transplantation experiments in three nude mice ( Supplementary Fig. 1d ), and the remaining parts for pathological and immunohistological analysis. The dissected tumours were confirmed as ADC without any p63-positive cells revealed by immunohistological and statistical analysis on serial sections. Interestingly, we were able to detect SCC derived from one out of three ADC with typical squamous morphology at later passage (passage 3), despite the initial Ttf1-expressing ADC pathology at early passages (passages 1–2) ( Supplementary Fig. 1e,f ). As in our previous study [16] , apart from those typical SCC we consistently observed a portion of mixed lesions with adenomatous and squamous pathologies in Kras / Lkb1 mice at 8–12 weeks post Ad-Cre treatment. These mixed lesions morphologically resembled the adenosquamous cell carcinoma observed in the clinic [8] , [9] , [10] , [11] , and were featured with a majority of p63-positive cells in proximity to SP-C-positive cells in a single tumour lesion ( Fig. 1e ). We henceforth arbitrarily defined these mixed lesions as mouse adenosquamous cell carcinoma (mAd-SCC), although most of them mainly contained squamous histology with a small part of ADC. At 8–10 weeks post Ad-Cre treatment, ~70% of squamous lesions were mAd-SCC. However, the percentage of mAd-SCC gradually decreased to ~30% at 10–12 weeks post Ad-Cre treatment, and to only 10% post an even longer time treatment (12–14 weeks). On the contrary, the percentage of typical SCC without mixed ADC pathology increased with time ( Fig. 1f ). Consistently, statistical analysis revealed that the average percentage of p63-positive cells progressively increased from 66 to 92% concomitantly with a decrease of average percentage of cells positive for SP-C from 34 to 8% in mAd-SCC from 8 to 12 weeks post Ad-Cre treatment ( Supplementary Fig. 1g,h ). Collectively, these data suggest that LKB1 -deficient ADC progressively transdifferentiate into SCC via a pathologically mixed intermediate as mAd-SCC. ADC from type II pneumocyte transdifferentiates into SCC Recent lineage-tracing experiments in mice have identified type II pneumocytes, Clara cells in the terminal bronchioles and putative bronchoalveolar stem cells as cells of origin fo r Kras -induced lung hyperplasia, and only type II cells appear to progress to ADC [19] . To further confirm ADC to SCC transdifferentiation in vivo , we performed lineage-tracing experiments in LKB1 -deficient mouse models. Based on the fact that mouse lung ADC is mainly derived from type II pneumocyte [4] , [5] , we constructed a mouse allele ( SP-C-CreERT2 ) using human SP-C promoter to drive CreERT2 expression specifically in this defined lineage [20] , [21] . We first examined the specificity as well as functionality of the SP-C promoter in SP-C-CreERT2/Rosa26R-LacZ mice. In the SP-C-CreERT2/Rosa26R-LacZ mice, we found that tamoxifen-induced LacZ expression from Rosa26 locus was specifically restricted to SP-C-positive type II pneumocytes, but not in basal cells that are Sox2-positive [22] ( Fig. 2a ; Supplementary Fig. 2a,b ); We then crossed SP-C-CreERT2 and SP-C-CreERT2 , Rosa26R-LacZ mice with Kras/Lkb1 mice to obtain a cohort of S P-C-CreERT2/ K ras/ L kb1 ( SKL ) and S P-C-CreERT2/ R osa26R-LacZ/ K ras/ L kb1 ( SRKL ) mice, respectively. In comparison with Kras/Lkb1 model, the SKL mice after tamoxifen administration displayed a slow but comparable kinetic of tumour progression ( Supplementary Fig. 2c ). At 4–8 weeks post tamoxifen administration, a large proportion of type II pneumocytes were targeted by CreERT2 activation and stained positive for SP-C with a progressive process from AAH, adenoma, to ADC, whereas no p63-positive SCC lesion was detectable yet ( Supplementary Fig. 2d,e ). As expected, lung ADC was detected with positive X-gal staining ( Supplementary Fig. 2f ), indicating that most if not all ADC in SKL model were derived from SP-C-positive lineages. At 9–12 weeks post tamoxifen administration, the number of ADC increased, and a few typical SCC began to appear ( Fig. 2b ). At a longer time (13–16 weeks) post tamoxifen administration, the number of SCC increased significantly while that of ADC decreased ( Fig. 2b ). The SCC was positive for X-gal staining, highlighting their primary origin of ADC ( Supplementary Fig. 2f ). Moreover, the SCC had larger tumour size than ADC ( Fig. 2c,d ), consistent with the observation from the Kras/Lkb1 mouse model ( Fig. 1c,d ). Further detailed analyses revealed that the ratio of mAd-SCC to SCC gradually decreased from 9 to 16 weeks post tamoxifen administration ( Supplementary Fig. 2g,h ). We further characterized the transdifferentiation process using p63 and SP-C immunohistostaining combined with statistical analyses on tumours from SKL mice at different time points. The average percentage of p63-positive cells progressively increased from 82 to 92% concomitantly with a decrease of average percentage of cells positive for SP-C from 18 to 8% in mAd-SCC from 9–12 to 13–16 weeks post tamoxifen treatment ( Supplementary Fig. 2i,j ), indicating the gradual progress of transdifferentiation from ADC into SCC through mAd-SCC as the intermediate. Together, our data from three different animal models consistently support de novo ADC to SCC transdifferentiation. 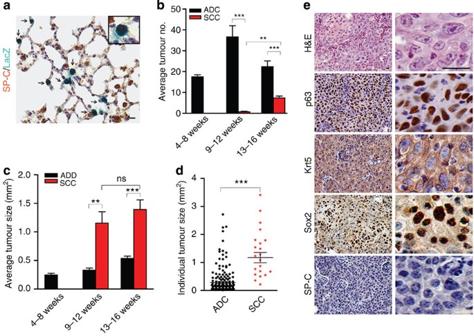Figure 2: Type II pneumocyte lineage-derived lung ADC withLkb1deficiency transdifferentiates into SCC. (a) Representative photos for SP-C and X-gal double staining in lung sections ofSP-C-CreERT2/Rosa26R-LacZmice at 2 weeks post tamoxifen administration. Scale bar, 10μm. (b,c) Quantification of average tumour number (b) and tumour size (c) per mouse for ADC and SCC inSP-C-CreERT2/Kras/Lkb1(SKL) mice at 4–8 weeks (n=8), 9–12 weeks (n=8), 13–16 weeks (n=10) post tamoxifen administration. Data are shown as mean±s.e.m.t-test, **P<0.01, ***P<0.001. (d) Quantification of individual tumour size for ADC and SCC inSKLmice at 12 weeks post tamoxifen administration (n=6). Data are shown as mean±s.e.m.t-test, ***P<0.001. (e) Representative SCC inSKLmice with haematoxylin and eosin staining and immunohistochemical staining for p63, Krt5, Sox2 and SP-C. Scale bar, 10 μm. Figure 2: Type II pneumocyte lineage-derived lung ADC with Lkb1 deficiency transdifferentiates into SCC. ( a ) Representative photos for SP-C and X-gal double staining in lung sections of SP-C-CreERT2/Rosa26R-LacZ mice at 2 weeks post tamoxifen administration. Scale bar, 10μm. ( b , c ) Quantification of average tumour number ( b ) and tumour size ( c ) per mouse for ADC and SCC in SP-C-CreERT2/Kras/Lkb1 ( SKL ) mice at 4–8 weeks ( n =8), 9–12 weeks ( n =8), 13–16 weeks ( n =10) post tamoxifen administration. Data are shown as mean±s.e.m. t -test, ** P <0.01, *** P <0.001. ( d ) Quantification of individual tumour size for ADC and SCC in SKL mice at 12 weeks post tamoxifen administration ( n =6). Data are shown as mean±s.e.m. t -test, *** P <0.001. ( e ) Representative SCC in SKL mice with haematoxylin and eosin staining and immunohistochemical staining for p63, Krt5, Sox2 and SP-C. Scale bar, 10 μm. Full size image ECM remodelling in ADC to SCC transdifferentiation To gain mechanistic insights into ADC to SCC transdifferentiation process, we performed bioinformatic analysis on the gene expression profiles of LKB1 -deficient mouse ADC and SCC from our previous study [16] , to search for those significantly deregulated signalling pathways. Notably, the 20 signalling pathways identified are mainly involved in cell–cell interaction and ECM remodelling process ( Fig. 3a and Supplementary Table 1 ). We then randomly selected and compared several established gene signatures related to these pathways [23] , [24] . Among these, there was an increase of genes associated with cell junctions in SCC relative to ADC, which include those participating in desmosome ( Pkp1 , Pkp3 , Dsc2 , Dsc3 , Dsg2 , Dsp , Jup and Perp ), tight junction ( Cldn4 , Cldn7 , Cldn8 and Cldn23 ) and gap junction ( Gjb2 and Gjb3 ) ( Fig. 3b and Supplementary Table 2 ). Besides, several genes involved in ECM degradation ( Mmp9 and Mmp14 ) were significantly upregulated in SCC, and certain matrix metalloproteinase (MMP) inhibitors ( Timp2 , Timp3 and Timp4 ) were downregulated ( Fig. 3b and Supplementary Table 2 ). In particular, several genes of collagen family essential for ECM homoeostasis were also robustly decreased in SCC ( Fig. 3b and Supplementary Table 2 ). Independent validation using real-time PCR analyses confirmed the changes of most gene signatures ( Supplementary Fig. 3 ). 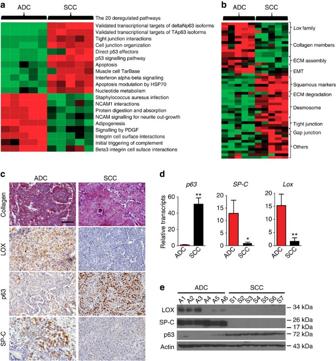Figure 3: Deregulation of Lox and ECM in lung SCC transdifferentiated from ADC withLKB1deficiency. (a,b) Heat maps showing significantly upregulated (red) and downregulated (green) pathways (a) and gene signatures (b) between ADC and SCC fromKras/Lkb1mice. (c) Representative photos showing Massons Trichrome staining of collagen as well as immunohistochemical staining for Lox, p63 and SP-C in lung ADC and SCC fromKras/Lkb1mice. Scale bar, 50 μm. (d) Real-time PCR detection of mRNA levels forp63,SP-CandLoxin lung ADC (n=8) and SCC (n=8) fromKras/Lkb1mice. Data are shown as mean±s.e.m.t-test, *P<0.05, **P<0.01. (e) Western blot detection of protein levels for p63, SP-C and Lox in lung ADC (n=6, A1–6) and SCC (n=7, S1–7) fromKras/Lkb1mice. Actin serves as control, see alsoSupplementary Fig. 9a. Figure 3: Deregulation of Lox and ECM in lung SCC transdifferentiated from ADC with LKB1 deficiency. ( a , b ) Heat maps showing significantly upregulated (red) and downregulated (green) pathways ( a ) and gene signatures ( b ) between ADC and SCC from Kras/Lkb1 mice. ( c ) Representative photos showing Massons Trichrome staining of collagen as well as immunohistochemical staining for Lox, p63 and SP-C in lung ADC and SCC from Kras/Lkb1 mice. Scale bar, 50 μm. ( d ) Real-time PCR detection of mRNA levels for p63 , SP-C and Lox in lung ADC ( n =8) and SCC ( n =8) from Kras/Lkb1 mice. Data are shown as mean±s.e.m. t -test, * P <0.05, ** P <0.01. ( e ) Western blot detection of protein levels for p63, SP-C and Lox in lung ADC ( n =6, A1–6) and SCC ( n =7, S1–7) from Kras/Lkb1 mice. Actin serves as control, see also Supplementary Fig. 9a . Full size image Even though the Kras activation and Lkb1 inactivation were initially engineered in our mouse models, it is unlikely to exclude the occurrence of new mutations in the mature tumours, which may confound our observation of transdifferentiation process. We then sequenced the genes of p53 , PIK3CA , p16 , Cul3 , Nrf2 , Keap1 and p19 in 4 lung ADCs and 4 SCCs derived from Kras/Lkb1 mice (primers are decribed in Supplementary Table 3 ), because the mutations of these genes have been reported in human lung SCC [25] . However, no mutation was detected for these genes in both ADC and SCC. LOX promotes ECM assembly by covalent intra- or inter-molecular crosslinking of collagen via oxidatively deaminating specific lysine and hydroxylysine residues in the telopeptide domains [26] . Elevated expression of LOX, frequently observed in several epithelial tumours, including breast cancer as well as head and neck cancer, promotes cancer progression and metastasis [27] , [28] , [29] . However, our bioinformatic analysis revealed that Lox was robustly downregulated in SCC relative to ADC in Kras/Lkb1 mice ( Fig. 3b and Supplementary Table 2 ). Consistent with less collagen deposition ( Fig. 3c ), we found that Lox mRNA levels decreased in SCC when compared with ADC ( Fig. 3d ). Indeed, expression of Lox could be detected in most of dissected ADC but not in SCC as shown by western blotting analysis ( Fig. 3e ). To determine whether such patterns of LOX expression and the collagen deposition are present in human lung cancer samples, we analysed 85 human lung ADCs and 85 SCCs on tissue microarray. Interestingly, we found that most of human lung SCCs showed low or negative Lox expression as well as collagen deposition compared with lung ADCs ( Supplementary Fig. 4 ). Studies using regular sequencing or deep sequencing of genomic DNA show that LKB1 inactivating mutations are frequently observed in ~20% of human ADC but only ~2% SCC [25] , [30] , [31] , [32] . Since LKB1 genetic alteration involves point mutation as well as exonic deletion, we have previously identified ~19% (8/42) of human lung SCC with LKB1 genetic alterations by the combination of direct sequencing and molecular analysis with multiplex ligation-dependent probe amplification (MLPA) analysis of genomic DNA [16] . Indeed, exonic deletion of LKB1 or even loss of whole gene allele cannot be detected by either regular sequencing or deep sequencing of genomic DNA due to the normal tissue contamination during the PCR process. 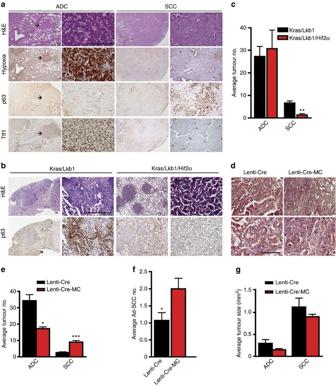Figure 4: Involvement of hypoxia and collagen deposition in ADC to SCC transdifferentiation. (a) Comparison of hypoxia levels in lung ADC and SCC fromKras/Lkb1mouse model. Scale bar, 150 μm. (b) Representative photos for haematoxylin and eosin and p63 immunohistochemical staining inKras/Lkb1andKras/Lkb1/Hif2amice at 10 weeks post Ad-Cre treatment, Scale bar, 150 μm. (c) Quantification of average tumour number per mouse for ADC and SCC fromKras/Lkb1mice (n=8) andKras/Lkb1/Hif2amice (n=7). Data are shown as mean±s.e.m.t-test, **P<0.01. (d) Massons Trichrome staining of lung ADC fromKras/Lkb1mice virally infected by either Lenti-Cre or Lenti-Cre-MC. Scale bar, 150 μm. (e,f) Quantification of average tumour number per mouse for ADC and SCC (e) and mAd-SCC (f) fromKras/Lkb1mice virally infected with Lenti-Cre (n=8) or Lenti-Cre-MC (n=7). Data are shown as mean±s.e.m.t-test, *P<0.05, ***P<0.001. (g) Quantification of average tumour size per mouse for ADC and SCC fromKras/Lkb1mice virally infected with Lenti-Cre (n=8) or Lenti-Cre-MC (n=7). Data are shown as mean±s.e.m. Using the same method, we analysed another ethnically different cohort with 101 Chinese lung SCC samples and identified ~13% (13 of 101) of Chinese squamous cell carcinoma with LKB1 exonic deletions plus 5% (5 of 101) patients harbouring LKB1 F354L mutation, which has been indicated as an inactivating mutation [33] , [34] (Supplementary Table 4). We next studied how Lox was downregulated in Lkb1 -deficient mouse SCC. We recently found that upregulated Lox expression through activation of mTOR–Hif1α signalling axis correlates with Lkb1 inactivation status and triggers excessive collagen deposition in Lkb1 -deficient lung ADC to enhance tumour cell proliferation and invasion [35] . We thus compared the hypoxia level in ADC and SCC and found the hypoxia level was dramatically decreased in SCC at 8 weeks post Ad-Cre treatment ( Fig. 4a ). To test whether the change of hypoxia level contributes to the ADC to SCC transdifferentiation, we crossed Hif2α mice with Kras/Lkb1 mice to functionally confirm the effect of hypoxia level on the transdifferentiation process [36] , [37] . After 10 weeks Ad-Cre treatment, Kras/Lkb1/Hif2α mice and Kras/Lkb1 mice were histopathologically and statistically analysed. Activation of Hif2α in Kras/Lkb1 mice dramatically inhibited the transdifferentiation process, as shown of the decrease of SCC number compared with control group ( Fig. 4b,c ). These data demonstrated that hypoxia deregulation play a causative role in the ADC to SCC transdifferentiation process. Figure 4: Involvement of hypoxia and collagen deposition in ADC to SCC transdifferentiation. ( a ) Comparison of hypoxia levels in lung ADC and SCC from Kras/Lkb1 mouse model. Scale bar, 150 μm. ( b ) Representative photos for haematoxylin and eosin and p63 immunohistochemical staining in Kras/Lkb1 and Kras/Lkb1/Hif2a mice at 10 weeks post Ad-Cre treatment, Scale bar, 150 μm. ( c ) Quantification of average tumour number per mouse for ADC and SCC from Kras/Lkb1 mice ( n =8) and Kras/Lkb1/Hif2a mice ( n =7). Data are shown as mean±s.e.m. t -test, ** P <0.01. ( d ) Massons Trichrome staining of lung ADC from Kras/Lkb1 mice virally infected by either Lenti-Cre or Lenti-Cre-MC. Scale bar, 150 μm. ( e , f ) Quantification of average tumour number per mouse for ADC and SCC ( e ) and mAd-SCC ( f ) from Kras/Lkb1 mice virally infected with Lenti-Cre ( n =8) or Lenti-Cre-MC ( n =7). Data are shown as mean±s.e.m. t -test, * P <0.05, *** P <0.001. ( g ) Quantification of average tumour size per mouse for ADC and SCC from Kras/Lkb1 mice virally infected with Lenti-Cre ( n =8) or Lenti-Cre-MC ( n =7). Data are shown as mean±s.e.m. Full size image As indicated by the association of the significantly deregulated pathways and gene signatures to ECM, we focused on the role of LOX in ECM remodelling, although intracellular roles of LOX were also documented [38] . To this, we infected Kras/Lkb1 mice with lentivirus carrying Cre recombinase with or without the dominant-negative minigene version of type I human procollagen (MC) that inhibits collagen maturation and deposition (Lenti-Cre and Lenti-Cre-MC) [39] , [40] , and analysed lung tumour formation at 13 weeks post treatment ( Supplementary Fig. 5a ) [41] , [42] . With a relatively slower progression pattern than Ad-Cre treatment, Lenti-Cre administration led to similar pathological phenotype, including ADC, mAd-SCC and typical SCC formation ( Supplementary Fig. 5b ). Lenti-Cre-MC infection reduced tumour collagen deposition and decreased the average number and size of lung ADC ( Fig. 4d,e,g ), confirming the positive role of collagen deposition in lung ADC progression [35] . On the contrary, the average number of SCC as well as Ad-SCC was increased by Lenti-Cre-MC infection without significant impact upon the average SCC size ( Fig. 4e–g ), indicating an enhanced ADC to SCC transdifferentiation. Together, these data suggest a role of Lox downregulation in the ADC to SCC transdifferentiation potentially through decreasing collagen deposition. Lox overexpression inhibits ADC to SCC transdifferentiation To explore the role of Lox-mediated ECM remodelling in ADC to SCC transdifferentiation, we first tested the effect of ectopic Lox expression upon this process. We infected Kras/Lkb1 mice with lentivirus carrying Cre recombinase with or without Lox expression (Lenti-Cre or Lenti-Cre-Lox), and compared the SCC formation at 13 weeks post treatment ( Fig. 5a ). Consistent with Ad-Cre treatment, Lenti-Cre administration led to similar pathological phenotype, including ADC, Ad-SCC and typical SCC formation. Lenti-Cre-Lox infection led to high expression of Lox and increased collagen deposition in lung tumours ( Fig. 5b ). Strikingly, only 27% (3/11) of mice in Lenti-Cre-Lox group developed SCC, in contrast to 91% (10/11) of mice in Lenti-Cre group with SCC post 13 weeks of viral treatment, indicating that the incidence of SCC formation was significantly inhibited by ectopic Lox expression. Indeed, most tumours in Lenti-Cre-Lox group were ADC and positive for SP-C staining ( Supplementary Fig. 6 ). Moreover, ectopic expression of Lox significantly decreased the number of SCC while increased that of ADC ( Fig. 5c,d ), but had little effect upon average tumour size of either subtype ( Fig. 5e ). These data demonstrated that ectopic Lox expression inhibits ADC to SCC transdifferentiation potentially through ECM remodelling. 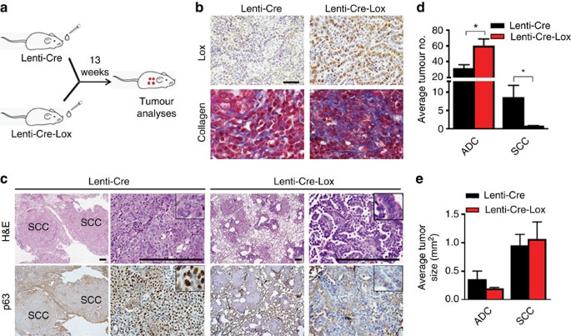Figure 5: Ectopic expression of lox inhibits ADC to SCC transdifferentiation. (a) Scheme of viral infection strategy for ectopic Lox expression inKras/Lkb1mouse model. (b) Lox immunohistochemical staining and Massons Trichrome staining in lung ADC inKras/Lkb1mice at 13 weeks post viral infection with Lenti-Cre or Lenti-Cre-Lox. Scale bar, 150 μm. (c) Representative photos for lung SCC formation and p63 immunohistochemical staining. Scale bar, 150 μm. (d,e) Quantification of average tumour number (d) and tumour size (e) per mouse for ADC and SCC fromKras/Lkb1mice virally infected with Lenti-Cre(n=11) or Lenti-Cre-Lox(n=11). Data are shown as mean±s.e.m.t-test, *P<0.05. Figure 5: Ectopic expression of lox inhibits ADC to SCC transdifferentiation. ( a ) Scheme of viral infection strategy for ectopic Lox expression in Kras/Lkb1 mouse model. ( b ) Lox immunohistochemical staining and Massons Trichrome staining in lung ADC in Kras/Lkb1 mice at 13 weeks post viral infection with Lenti-Cre or Lenti-Cre-Lox. Scale bar, 150 μm. ( c ) Representative photos for lung SCC formation and p63 immunohistochemical staining. Scale bar, 150 μm. ( d , e ) Quantification of average tumour number ( d ) and tumour size ( e ) per mouse for ADC and SCC from Kras/Lkb1 mice virally infected with Lenti- Cre ( n =11) or Lenti- Cre - Lox ( n =11). Data are shown as mean±s.e.m. t -test, * P <0.05. Full size image Lox inhibition promotes ADC to SCC transdifferentiation We then performed pharmacological targeting of Lox enzymatic activity to mimic Lox downregulation and investigated its impact upon this process. We utilized β-aminoproprionitrile (BAPN), a well-documented chemical that directly binds to the active site of LOX and irreversibly inhibits its enzymatic activity to affect the crosslinking of collagen molecules [27] , [43] , [44] , [45] . In our previous study, we found that BAPN treatment for 8 weeks significantly inhibited the progression of Kras/Lkb1 ADC [35] . In this study, we herein performed a shorter term of BAPN treatment (4 weeks) on Kras/Lkb1 mice, with a focus on the transdifferentiation process ( Fig. 6a ). As expected, BAPN treatment significantly decreased mouse serum Lox enzymatic activity and collagen deposition in lung ADC ( Supplementary Fig. 7a,b ). Strikingly, we found that a high percentage of BAPN-treated mice (86%, 12/14) developed SCC, in contrast to only 17% (3/18) of control mice with SCC ( Table 1 ). The average number of SCC in BAPN-treated mice significantly increased with a concomitant decrease of ADC number ( Fig. 6b,c ). Moreover, BAPN treatment increased the average number of mAd-SCC ( Fig. 5d ), indicating the acceleration of the transdifferentiation process. This is consistent with the statistical analyses of the percentage of SP-C and/or p63-positive cells ( Supplementary Fig. 7c,d ). However, we observed no significant effect of BAPN treatment upon the average size of either tumour subtype ( Fig. 6e,f ). The essential role of Lox in ADC to SCC transdifferentiation was further supported by BAPN treatment in SKL mice, with lung tumours from defined cell lineage. The incidence of SCC formation was dramatically increased by BAPN treatment, from 15% (3/20) to 60% (12/20) ( Supplementary Fig. 7f–i , Table 1 ). 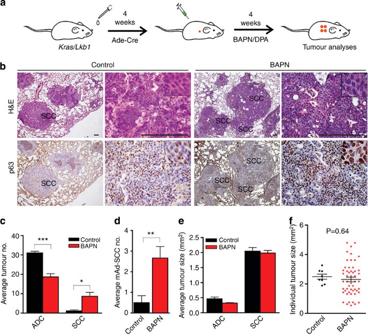Figure 6: Pharmacological inhibition of Lox enzymatic activity promotes ADC to SCC transdifferentiation. (a) A scheme for BAPN and DPA treatment inKras/Lkb1mice. (b) Representative photos for haematoxylin and eosin and p63 immunohistochemical staining inKras/Lkb1mice treated with BAPN or saline. Scale bar, 150 μm. (c,d) Quantification of average tumour number per mouse for ADC and SCC (c) and mAd-SCC (d) fromKras/Lkb1mice treated with BAPN (n=14) or saline (n=18). Data are shown as mean±s.e.m.t-test, *P<0.05, **P<0.01, ***P<0.001. (e,f) Quantification of average tumour size per mouse for ADC and SCC (e) and individual tumour size for SCC (f) fromKras/Lkb1mice post BAPN (n=14) or saline (n=18) treatment. Data are shown as mean±s.e.m.t-test, *P<0.05, **P<0.01, ***P<0.001. Figure 6: Pharmacological inhibition of Lox enzymatic activity promotes ADC to SCC transdifferentiation. ( a ) A scheme for BAPN and DPA treatment in Kras/Lkb1 mice. ( b ) Representative photos for haematoxylin and eosin and p63 immunohistochemical staining in Kras/Lkb1 mice treated with BAPN or saline. Scale bar, 150 μm. ( c , d ) Quantification of average tumour number per mouse for ADC and SCC ( c ) and mAd-SCC ( d ) from Kras/Lkb1 mice treated with BAPN ( n =14) or saline ( n =18). Data are shown as mean±s.e.m. t -test, * P <0.05, ** P <0.01, *** P <0.001. ( e , f ) Quantification of average tumour size per mouse for ADC and SCC ( e ) and individual tumour size for SCC ( f ) from Kras/Lkb1 mice post BAPN ( n =14) or saline ( n =18) treatment. Data are shown as mean±s.e.m. t -test, * P <0.05, ** P <0.01, *** P <0.001. Full size image Table 1 Incidence of SCC formation in different mouse models after lox inhibition. Full size table We further used another chemical, D -penicillamine (DPA) to inhibit Lox enzymatic activity. Different from BAPN, DPA inhibits Lox function by chelating its cofactor copper [46] . DPA treatment also resulted in a significant decrease of serum Lox enzymatic activity and collagen deposition in lung ADC ( Supplementary Fig. 7a,b ). We observed a promoter effect of DPA upon ADC to SCC transdifferentiation, as 71% (10/14) of Kras/Lkb1 mice harboured SCC post 4 weeks of DPA treatment ( Table 1 ). The number of ADC decreased significantly, while the number of SCC as well as mAd-SCC increased dramatically ( Supplementary Fig. 7j,k ). No obvious change was found on the tumour size of either ADC or SCC after DPA treatment ( Supplementary Fig. 7l,m ). Importantly, detailed immunohistological and statistical analyses revealed a decrease of cell proliferation with a concomitant increase of cell apoptosis in certain ADC from Kras/Lkb1 mice after BAPN or DPA treatment in comparison with those from control group ( Supplementary Fig. 7n–q ). However, no significant difference of either cell proliferation or apoptosis was observed in SCC with or without Lox inhibition. Even with BAPN or DPA treatment, these SCC still maintained a high rate of cell proliferation and a low rate of apoptosis ( Supplementary Fig. 7n–q ). These data reveal the different response of lung SCC and ADC towards Lox inhibition and highlight an important outcome of ADC to SCC transdifferentiation in drug resistance development. ECM remodelling regulates transdifferentiation through p63 To further dissect the downstream effector of Lox-mediated ECM remodelling in ADC to SCC transdifferentiation, we performed a short term of BAPN treatment on Kras/Lkb1 mice. At as early as 2 weeks post BAPN treatment, apart from few typical SCC lesions, we observed several lesions with typical ADC pathology but with a few cells positive for p63 staining ( Fig. 7a ). In addition, increased expression of p63 was also detected in BAPN-treated subcutaneous tumours from human NSCLC cell line A549 in nude mice ( Fig. 7b ). P63 , especially the delta-N isoforms ( DNp63 ) act as master lineage survival oncogenes of SCC, and play essential roles in epithelial stratification and squamous cell survival [47] , [48] . We thus postulated that p63 activation is an essential early step of the squamous transdifferentiation. Aiming to search for potential p63 upstream regulators, we searched the literature and then comparatively analysed mouse lung ADC and SCC expression profiles, and identified a list of SCC signature genes including Brf2 , c-Myc , Dlx5 , Klf5 , Oct1 , Sccro and Trim29 . Consistent with previous studies [49] , [50] , [51] , [52] , expression of these genes was significantly higher in mouse lung SCC than ADC ( Supplementary Fig. 8a ), and a short term of BAPN treatment increased the expression of most genes ( c-Myc , Dlx5 , Oct1 , and Sccro ) in LKB1 -deficient mouse lung ADC ( Fig. 7c ). Interestingly, individual expression of most genes ( Brf2 , c-Myc , Dlx5 , Klf5 , Sccro and Trim29 ) upregulated p63 transcription in human NSCLC cell lines ( Fig. 7d ). Since the Kras/p53 mouse model only produces lung ADC [12] , we next tested whether ectopic p63 overexpression can drive de novo squamous transdifferentiation from ADC in Kras/p53 mouse model. We then established primary cell lines from dissected Kras/p53 lung ADC, and performed DNp63a overexpression in vitro followed by lung-seeding assays in nude mice. Our data showed that transient DNp63a expression in Kras/p53 cells activated Krt5 and Krt14 expression ( Supplementary Figs 8b,c and 9b ), and cells with stable DNp63a expression showed distinct morphologies from parental cells ( Supplementary Fig. 8d ). Notably, apart from certain known p63 target genes ( Krt5 and Krt14 ), DNp63a -expressing Kras/p53 cells also expressed a series of genes previously identified as SCC signature genes ( Fig. 7e ). In the lung-seeding assays in nude mice, several tumours derived from DNp63a -expressing Kras/p53 ADC cells were consistently found with SCC-like pathology, while parental cells only gave rise to ADC pathology. Although stained positive for squamous marker Krt5, these SCC-like tumours still expressed ADC marker Ttf1, indicating a squamous transdifferentiation process albeit incomplete ( Fig. 7f ). These data demonstrate that ectopic expression of lineage survival oncogene DNp63a is able to partially drive de novo ADC to SCC transdifferentiation. 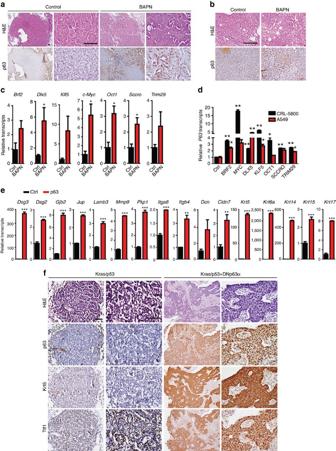Figure 7: Lox inhibition activates p63 to promote ADC to SCC transdifferentiation. (a) Representative photos for haematoxylin and eosin staining and p63 immunohistochemical staining of lung tumours fromKras/Lkb1mice treated with BAPN or saline for 2 weeks. Scale bar, 150 μm. (b) Representative photos for haematoxylin and eosin staining and p63 immunohistochemical staining on tumours derived from A549 xenografts in nude mice with or without BAPN treatment. Scale bar, 150 μm. (c) Real-time PCR analysis of relative expression of SCC signature genes in lung ADC fromKras/Lkb1mice treated with BAPN (n=5) or saline (n=7) for 2 weeks. Data are shown as mean±s.e.m.t-test, *P<0.05, **P<0.01, ***P<0.001. (d) Real-time PCR analysis shows that the SCC signature genes can transcriptionally upregulatep63in human NSCLC cell lines A549 and CRL5800 (three replicates for each sample). Data are shown as mean±s.e.m.t-test, *P<0.05, **P<0.01, ***P<0.001. (e) Real-time PCR analysis of relative expression of a serial of SCC signature genes inKras/p53ADC cells with or without ectopic p63 expression (three replicates for each sample). Data are shown as mean±s.e.m.t-test, *P<0.05, **P<0.01, ***P<0.001. (f) Representative histology, immunohistochemical staining for p63, Krt5 and Ttf1 in lung tumours derived fromKras/p53ADC cells with or without ectopic DNp63α expression in nude mice lung seeding assay. Scale bar, 150 μm. Figure 7: Lox inhibition activates p63 to promote ADC to SCC transdifferentiation. ( a ) Representative photos for haematoxylin and eosin staining and p63 immunohistochemical staining of lung tumours from Kras/Lkb1 mice treated with BAPN or saline for 2 weeks. Scale bar, 150 μm. ( b ) Representative photos for haematoxylin and eosin staining and p63 immunohistochemical staining on tumours derived from A549 xenografts in nude mice with or without BAPN treatment. Scale bar, 150 μm. ( c ) Real-time PCR analysis of relative expression of SCC signature genes in lung ADC from Kras/Lkb1 mice treated with BAPN ( n =5) or saline ( n =7) for 2 weeks. Data are shown as mean±s.e.m. t -test, * P <0.05, ** P <0.01, *** P <0.001. ( d ) Real-time PCR analysis shows that the SCC signature genes can transcriptionally upregulate p63 in human NSCLC cell lines A549 and CRL5800 (three replicates for each sample). Data are shown as mean±s.e.m. t -test, * P <0.05, ** P <0.01, *** P <0.001. ( e ) Real-time PCR analysis of relative expression of a serial of SCC signature genes in Kras / p53 ADC cells with or without ectopic p63 expression (three replicates for each sample). Data are shown as mean±s.e.m. t -test, * P <0.05, ** P <0.01, *** P <0.001. ( f ) Representative histology, immunohistochemical staining for p63, Krt5 and Ttf1 in lung tumours derived from Kras / p53 ADC cells with or without ectopic DNp63α expression in nude mice lung seeding assay. Scale bar, 150 μm. Full size image Phenotypic plasticity and functional heterogeneity are important features of tumours arising in various organs including the lung [25] , [53] , [54] . Dissecting the potential phenotypic plasticity and dynamic lineage correlation between tumour subtypes would enable a better understanding of tumourigenesis and the development of effective cancer therapeutic strategies. Recent study showed that the glioblastoma stem cells are able to transdifferentiate into endothelial cells [55] , [56] . The histopathological heterogeneity of lung cancer has been established, and the phenotypic plasticity between the tumour subtypes represents one of the unsolved questions. Indeed, one recent study has revealed the genotypic and histological transition of EGFR-mutant NSCLC into SCLC after targeted therapy [57] . Notably, the transition from neuroendocrine to mesenchymal phenotype could also be achieved by ectopic expression of oncogenic Ras V12 in SCLC [58] . However, the linage transition of ADC and SCC remains unknown. It is generally accepted that Kras -mutant ADC originates mainly from the lineage of type II pneumocytes with a stepwise progression from AAH to Adenoma, and then to ADC [3] , [41] , [59] , while lung SCC potentially have different cells of origin, possibly the basal cells [4] . Through detailed monitoring of tumour progression patterns in three different mouse models, we have here discovered a previously unexpected phenotypic plasticity of lung ADC: lung ADC with LKB1 deficiency can progressively transdifferentiate into SCC. Our data suggest that the majority if not all of the cells in ADC with LKB1 deficiency have the ability to transit to SCC. Moreover, the robust and systematic transdifferentiation process occurs in a stage-specific manner, different from traditional cancer stem cell theory in which a minor cell population, such as glioblastoma stem cells, was conferred with the phenotypic plasticity [55] , [56] . The transition is also different from the metaplasia through cell replacement as seen in PTEN -deficient pancreatic ADC development in mice [60] . Indeed, although we observed a statically significant difference of cell proliferating rate between ADC and SCC, these ADC cells still keep proliferating despitea lower rate than SCC cells. In line with this, we have identified the mixed pathology mAd-SCC as the intermediate for this transition process. This work proves the existence of lung ADC to SCC transdifferentiation in de novo mouse models, highlighting the phenotypic plasticity of lung ADC with LKB1 deficiency. Initial analyses of gene signatures for cell junctions and ECM homoeostasis, as wells as differential collagen deposition between ADC and SCC, have indicated that LKB1 -deficient ADC might depend more on ECM for survival and proliferation while SCC depends more on cell–cell interactions instead. Indeed, inhibition of collagen crosslinking by pharmacologically targeting Lox significantly suppresses ADC growth but has little effect upon SCC. Thus, the different extents to which ADC and SCC depend on ECM may reflect their differential sensitivity to ECM perturbation. Beyond this, we have established an important regulatory pathway for ECM in shaping phenotypic plasticity of lung ADC with LKB1 deficiency: At the early stage, loss of the tumour suppressor LKB1 promotes ADC progression partly through Lox [35] ; as the tumours grow up, Lox reduction following reduced hypoxia level would lead to ECM remodelling, which then results in the dramatic change so that the ADC cells might robustly and systematically transit to SCC. The transdifferentiation process would enable LKB1 -deficient ADC to overcome the stress derived from ECM deficiency so that the resultant SCC can keep growing at a high proliferation rate. Moreover, more stress would be accumulated in LKB1 -deficient ADC as they grow bigger. This may explain why we always observed SCC with a large tumour size, even at their initial appearances. A future challenge will be to decipher the identity of stress and other potential mechanisms to unveil the comprehensive molecular and cellular events in modulating ADC to SCC transdifferentiation. Our previous study suggested the LKB1 modulates lung tumour initiation, differentiation and metastasis possibly through independent mechanisms [16] . Consistently, ADC metastasis was only observed after 10 weeks post Ad-Cre treatment, while ADC to SCC transdifferentiation was observed at 8 weeks post Ad-Cre treatment. We reason the phenotypic transition occurs earlier than metastasis, and these two might be separate events during tumour progression. Together with our previous findings [35] , we unveil the dual function of Lox in LKB1 -deficient lung ADC, one hand to promote ADC progression and metastasis [35] , the other hand to inhibit ADC to SCC transdifferentiation via ECM remodelling (the present study). Notably, Lox enzymatic inhibition promotes LKB1 -deficient ADC transdifferentiation into SCC, which then becomes insensitive to Lox inhibition. Different from previously established molecular mechanisms involved in drug resistance development, this may represent a unique and novel mechanism for escaping drug treatment at the cellular level. Although this possibility remains to be tested clinically, our study might provide helpful insights into therapeutic strategy development for lung ADC in which somatic LKB1 mutations are highly prevalent. Mouse colony and tumour analyses Kras G12D /p53 L/L ( Kras/p53 ), Kras G12D /Lkb1 L/L ( Kras/Lkb1 ), and Rosa26-LacZ mice were originally provided by T. Jacks (Cambridge, MA), R. DePinho (Boston) and L. Cheng (Shanghai), respectively. All mice were housed in a pathogen-free environment at Shanghai Institute of Biochemistry and Cell Biology and treated in accordance with protocols approved by the Institutional Animal Care and Use Committee of the Shanghai Institute of Biochemistry and Cell Biology, Chinese Academy of Sciences. To make the SP-C-CreERT2 transgenic mice, a DNA fragment containing CreERT2-coding region plus the SV40 poly A was ligated to the 3.7-kb region of the human SP-C promoter [20] , and then microinjected into FVB/N blastocysts as described [61] . Progeny were screened using Southern blot and confirmed by PCR strategy. The Kras/Lkb1 mice were treated with a low dosage of Ade-Cre (2 × 10 6 PFU), 60% lower than the original dosage used in this model [16] , or Lentivirus (2 × 10 6 PFU) at 6–8 weeks of age via nasal inhalation as previously described [3] , [16] , [35] . Histological examinations were performed by the pathologist Dr Yingyong Hou from Zhongshan Hospital in Fudan University. For SP-C-CreERT2/Kras/Lkb1 ( SKL ) or SP-C-CreERT2/Rosa26R-LacZ/Kras/Lkb1 ( SRKL ) mouse models, tamoxifen in sunflower oil (40 mg kg −1 ) were given to male mice at 6–8 weeks of age via intraperitoneal injection every other day for five continuous doses. For pharmacological treatment in Kras/Lkb1 mice, either BAPN (100 mg kg −1 ), DPA (150 mg kg −1 ) or saline were given to mice at 4 weeks post Ad-Cre treatment via intraperitoneal injection daily for 4 weeks. The SKL and SRKL mice at 6 weeks post tamoxifen treatment were also administrated with BAPN for another 3 weeks. For hypoxia probe treatment, mice were administrated with hypoxia probe solution at a dosage of 1.5 mg per mouse and 60 minutes later, the lungs were fixed with 4% paraformaldehyde for the preparation of routine paraffin section. After the deparaffinization and hydration, the sections were incubated with 3% H 2 O 2 in distilled water and then in 10 mM Citrate (pH=6) for antigen retrieval. The primary antibody (FITC-MAb1) and the secondary antibody (HRP linked to rabbit anti-FITC IgG) were added and incubated at room temperature for 30 min respectively. Then DAB reaction, dehydration and mounting were performed as usual. All mice were then killed for gross inspection and histopathological examination. Tumour number was counted under microscope and tumour size was analysed using Image J software [35] , [61] . Nude mice experiments Human NSCLC cell lines A549 and CRL5800 were obtained from ATCC. Six-week-old male nude mice with BALB/c genetic backgroud were used in the experiments. All mice were housed in a pathogen-free environment at Shanghai Institute of Biochemistry and Cell Biology and treated in strict accordance with protocols approved by the Institutional Animal Care and Use Committee of the Shanghai Institute of Biochemistry and Cell Biology, Chinese Academy of Sciences. For serial transplant experiment, three primary Kras/Lkb1 ADCs dissected from mice at 6 weeks post Adeno-Cre infection were divided into two parts repectively: one part was homogenated and subcutaneously injected into the nude mice ( n =3), and the other part was used for pathological inspection. Once the tumours grew to 3–5 mm in diameter (at least 1 month) in nude mice (passage 1), these tumours were then dissected for continuous subcutaneous xenografts for another two passages (the average duration for the second and third passage is ~3 weeks). The pathology was inspected for each passage. A549 cells were subcutaneously injected into nude mice (5 × 10 6 cell per mouse) and BAPN (100 mg kg −1 ) or saline were given to mice 1 month later via intraperitoneal injection daily for 4 weeks. For lung seeding assay, Kras/p53 cells were inoculated into nude mice (2 × 10 6 cell per mouse) via tail vein injection, BAPN (100 mg kg −1 ) or saline were given to mice 1 month later via intraperitoneal injection daily for 4 weeks. The tumours were harvested for histopathological analysis and examined by a pathologist. Histology and immunohistochemistry Lungs from male and female mice were inflated with 1 ml 4% paraformaldehyde, fixed overnight and dehydrated in ethanol, embedded in paraffin, sectioned at 5 μm followed by staining with haematoxylin and eosin. Immunohistochemistry was performed as previously described [16] , [35] . The following antibodies were used: SP-C (AB3786, Chemicon; 1:2,000), Krt5 (BS1280, Bioworld, 1:200, 10 ng μl −1 ), p63 (SC-8431, Santa Cruz, this antibody specifically recognizes DNp63; 1:200, 1 ng ul −1 ), Sox2 (AB5603, Chemicon; 1:1,000, 1 ng μl), LOX (L4669, Sigma, 1:800, 1.25 ng μl −1 ), Ttf1 (5883-1, EPITOMICS; 1:500), Beta Galactosidase (ab9631, Abcam; 1:200). For β-galactosidase staining, mouse lungs were isolated and immediately incubated for 2 h in a 20-fold volume of ice-cold fixative (1% formaldehyde, 0.2% gluteraldehyde and 0.02% NP40 in PBS) at 4°C on a rolling platform. The fixative was removed and the tissues were washed twice in PBS for 20 min at room temperature. The galactosidase substrate (5 mM K 3 Fe (CN)6, 5 mM K 4 Fe (CN)6, 2 mM MgC l2 , 0.02% NP40, 0.1% sodium deoxycholate and 1 mg ml −1 X-gal in PBS) was then added and the tissues were incubated in the dark overnight. The stained tissues were transferred to tissue cassettes and fixed overnight and dehydrated in ethanol, embedded in paraffinand then sectioned at 5 μm for the following haematoxylin and eosin staining and immunohistochemical staining [62] . LOX enzymatic activity assay Mouse sera were collected for LOX enzymatic activity assessment [35] . Briefly, samples were prepared in a final volume of 1 ml containing 1.2 M urea (Amresco), 0.05 M sodium borate (Sigma, pH 8.2), 0.1 units per ml of horseradish peroxidase (Fluka), 50 μM Amplex Red (Invitrogen) and 10 mM 1, 5-diaminopentane (Sigma-Aldrich) and were incubated at 37 °C for 1 h. Fluorescence was measured using a Hitachi F-2000 fluorescence spectrophotometer. Parallel assays were prepared with 500 μM BAPN to completely inhibit the activity of LOX. The LOX activities were calculated as the increase in fluorescent units above the BAPN controls. Establishment of primary mouse tumour cell line Kras/p53 mice (male and female at 6–8 weeks of age) were treated with Ade-Cre (2 × 10 6 PFU) via nasal inhalation. Tumours were dissected after 10 weeks virus infection and cut into small pieces and cultured in DMEM (Hyclone) supplemented with 10% FBS (Biochrom). The medium was changed every other day until cells outgrew and stable cell lines were formed. Human lung cancer specimens collection Human lung cancer specimens were collected with the approval by the institutional review board of Shanghai Cancer Hospital, Fudan University, Shanghai, China. All patients gave written informed consent. Samples were snap-frozen in liquid nitrogen at the time of resection and stored at −80 °C until use. All cases were re-reviewed by pathologists for confirmation of tumour histology and tumour content. In the present study, 101 human lung SCC samples were used for exon sequencing and MLPA experiments as described previously [16] . Human tissue microarray sections containing 85 lung ADCs and 85 lung SCCs were immunohistochemically stained with an anti-Lox antibody and performed with Massons Trichrome staining for collagen deposition detection. Lentivirus production and infection The ORFs of Lox and DNp63a were amplified from mouse tumour cDNAs, and ligated into expression vectors pCDH-EF1-Puro (Systems Biosciences) or pCDH-EF1-Cre (adapted vector for Lox expression in vivo ). The production of lentivirus supernatant was described previously [35] , [41] . The human NSCLC cell lines A549 and CRL5800 (ATCC) were maintained in RPMI1640 (Hyclone) supplemented with 10% FBS (Biochrom). For transient overexpression, trypsinized cells were first incubated with virus supernatant (1:1 in volume) in a six-well plate (Corning) for 24 h, then cultured in fresh medium for another 24 h, and harvested for analysis. For stable overexpression of DN p63a , Kras/p53 ADC cells infected with virus were persistently cultured in medium with puromycin (2 μg ml −1 , Sigma) until lung seeding assays. Western blotting and real-time PCR analyses Lung tumours (≥2 mm in diameter) were freshly dissected from male and female Kras/Lkb1 mice at 8–10 weeks post Ad-Cre treatment. These tumours were immediately cut into several pieces, one piece was used for HE and IHC inspection, and the rest pieces were snap-frozen separately for western blotting and real-time PCR analyses. Western blot assays were performed as previously described with antibodies against p63 (SC-8431, Santa Cruz, this antibody specifically recognizes DNp63; 1:200, 1 ng μl −1 ), Lox (L4669, Sigma; 1:800, 1.25 ng μl −1 ), SP-C (AB3786, Chemicon; 1:2,000) and Actin (C-1, Santa Cruz; 1:2,000, 0.1 ng μl −1 ). Total RNA and genomic DNA were prepared as previously described [35] . Total RNA was retrotranscribed into first-strand cDNA using RevertAid First Strand cDNA Synthesis Kit (Fermentas). The cDNAs were then used for real-time PCR on a 7500 Fast Real-Time PCR System (Applied Biosystems) using SYBR-Green Master PCR mix (Toyobo). β-actin served as internal control. The primers for PCR were summarized in Supplementary Information ( Supplementary Table 5 ). Microarray data analysis Gene expression data (GEO accession: GSE6135 ) generated in the previous study was prefiltered using low stringency, pre-defined criteria: probe set intensity (>32 in all samples) and dynamic variation (more than twofold over the entire sample set) [16] . After filtering, multiple probe sets that presented the same genes were collapsed by taking the median value for that gene per array yielding 3,275 unique genes, on which two-way hierarchical clustering was performed. Gene expression microarray data were pre-processed with the RMA algorithm [63] , [64] . To identify pathways altered in each sample, we first constructed a virtual reference sample by taking the median across all samples, and then compared each sample with this reference to obtain twofold up- and downregulated genes, which were further tested against a catalogue of biological pathways with Fisher’s Exact Test. The pathways were collected from four public databases: KEGG ( www.genome.jp/kegg ), Reactome ( www.reactome.org ), PID ( pid.nci.nih.gov ) and Wikipathways ( wikipathways.org ). Pathways with <15 genes or >500 genes were excluded for analyses. For each pathway, we calculated its enrichment significance in both up- and downregulated genes in the i th sample, termed as and , respectively. In order to find pathways with expression patterns indicative of sample classes, here ADC and SCC, we summarized for each pathway k an SL (signed minus log) score defined as, where θ is 1 if and 0 otherwise. Pathways showing poor enrichment across samples (insignificant in more than half samples) were not included for further analyses. We used the k-Nearest Neighbour (k-NN) method (ties broken randomly) with leave-one-out cross validation to measure the accuracy of a pathway in classifying samples. Note k was always optimally chosen by maximizing the prediction accuracy. To achieve robust outcomes, we replicated the procedure for a number of times (100 here) and took the average accuracy as the final measure. Pathways with 100% average accuracy were chosen for further consideration. In the pathway-level heat map, colours were assigned according to the SL i , k scores, whereas in the gene-level heat map, they were assigned according to gene-wise standardized expressions. Statistical analysis Differences were compared using two-tailed Student’s t -test. P -value <0.05 was considered statistically significant. All analyses were performed with SPSS 16.0 (SPSS). How to cite this article: Han, X. et al. Transdifferentiation of lung adenocarcinoma in mice with Lkb1 deficiency to squamous cell carcinoma. Nat. Commun. 5:3261 doi: 10.1038/ncomms4261 (2014).